Fast growth of large-grain and continuous MoS2films through a self-capping vapor-liquid-solid method Most chemical vapor deposition methods for transition metal dichalcogenides use an extremely small amount of precursor to render large single-crystal flakes, which usually causes low coverage of the materials on the substrate. In this study, a self-capping vapor-liquid-solid reaction is proposed to fabricate large-grain, continuous MoS 2 films. An intermediate liquid phase-Na 2 Mo 2 O 7 is formed through a eutectic reaction of MoO 3 and NaF, followed by being sulfurized into MoS 2 . The as-formed MoS 2 seeds function as a capping layer that reduces the nucleation density and promotes lateral growth. By tuning the driving force of the reaction, large mono/bilayer (1.1 mm/200 μm) flakes or full-coverage films (with a record-high average grain size of 450 μm) can be grown on centimeter-scale substrates. The field-effect transistors fabricated from the full-coverage films show high mobility (33 and 49 cm 2 V −1 s −1 for the mono and bilayer regions) and on/off ratio (1 ~ 5 × 10 8 ) across a 1.5 cm × 1.5 cm region. Apart from graphene, transition metal dichalcogenides (TMDs) with atomic thickness are the most renowned two-dimensional (2D) materials because of their excellent electrical and optical properties [1] , [2] , [3] , [4] , [5] , [6] . Their robust physical properties in atmosphere enable their practical applications in novel optoelectronic devices [7] , [8] . For electronics, TMDs with atomic thickness, which inherently have no surface dangling bonds, are immune to mobility degradation and short channel effects in contrast to conventional three-dimensional materials, such as Si and GaAs [9] , [10] , [11] . Such materials have layer-dependent bandgaps from near infrared to visible regions [12] , [13] , and thus, TMDs are favorable for energy or optical applications [7] , [8] , [14] , [15] . Furthermore, the difference between Berry curvature at the K and K′ valleys of monolayer TMDs generates new opportunities for valleytronics [16] , [17] . Despite these remarkable properties, TMDs still have limitations arising from spatial nonuniformity. Therefore, the fabrication of high-quality and large-grain films is thus crucial for TMDs. Currently, chemical vapor deposition (CVD) is the most recognized method for producing high-quality monolayer TMDs because of its low cost and scalability [18] , [19] , [20] , [21] , [22] . Conventional CVD methods of TMD fabrication are based on the reaction of gas-phase chalcogens (e.g., S and Se) and metal oxides (e.g., MoO 3 and WO 3 ) [18] , [19] , [20] , [21] , [22] . Generally, in gas-phase reactions, the grain size of TMDs is limited by the high nucleation density and typically is <500 µm. Recently, researchers have used various methods, which include fabricating at a high temperature [23] , inserting diffusion barriers [24] , and using an extremely small amount of precursors [25] , to reduce nucleation density and to increase the surface diffusion length for growing large TMD crystals. These methods can produce comparatively large crystals but considerably reduce the coverage of TMD crystals [25] , which hinders their practical applications. For bulk materials, Czochralski [26] , [27] method enables the production of a single-crystal ingot with a diameter of up to 300 mm by vertically pulling a solid seed crystal from a liquid source [28] . This method provides the unprecedentedly high uniformity of conventional bulk materials at an ultra-large scale. Moreover, a liquid source can more easily dissolve other solid dopants than a gas–gas reaction [29] . Therefore, it is desirable to grow solid crystals from liquid sources. For the growth of TMDs, Li et al. recently proposes the vapor–liquid–solid (VLS) reaction for fabricating high-quality MoS 2 nanoribbons from a liquid precursor on a sodium chloride (NaCl) single crystal [30] . First, NaCl reacts with MoO 3 to form a eutectic compound (Na 2 Mo 2 O 7 ), which has a relatively lower melting point and exists in a liquid phase under growth conditions (generally 700–800 °C). Second, the sulfur vapor is rapidly dissolved into the liquid and reacts to form a solid-state monolayer MoS 2 on NaCl. However, because of the low wettability between the NaCl and liquid Na 2 Mo 2 O 7 droplets, this method can only generate MoS 2 nanoribbons, which considerably limits its application. This problem can be solved by growing on other substrates with a better wettability [31] . Herein, a self-capping vapor–liquid–solid (SCVLS) reaction, which can grow large single crystals and full-coverage TMD films, is proposed. A solid precursor comprising ultra-thin MoO 3 , SiO 2 , and NaF layers was used for the controllable eutectic reaction of MoO 3 and NaF at high temperature. The as-formed eutectic liquid (Na 2 Mo 2 O 7 ) rose to the surface and was sulfurized into MoS 2 seeds. These seeds, acted as a self-capping layer, redirected the rising liquid into a horizontal direction. The residual liquid was continuously pushed along the growth direction and eventually sulfurized to form new MoS 2 at the edge of the MoS 2 seeds. This growth mechanism enables fabrication of ultra-large (~1.1 mm) single crystals. Moreover, continuous large-area MoS 2 film with large-grain size (~450 µm) can also be fabricated using thicker precursor. By controlling the kinetic factors of this reaction, the layer number can be controlled and large bilayer MoS 2 (~200 µm) can be achieved. In this study, the quality and uniformity of MoS 2 grown using this method are evaluated through electron microscopy, optical spectroscopy, and electrical measurements. For electrical measurements, both mono- and bilayer MoS 2 field-effect transistors (FETs) show high mobility (33 and 49 cm 2 V −1 s −1 ), large on/off ratio (5 × 10 8 ), and high current density (up to 230 and 390 µA µm −1 ). The large-grain, continuous film exhibits high performance across a 1.5 ×1.5 cm area, making the SCVLS method promising for practical applications. Material synthesis and growth mechanism Figures 1a and S1 show that a smooth MoO 3 layer was grown on c-plane sapphire through plasma-enhanced atomic layer deposition (PEALD). SiO 2 and NaF layers were stacked on top of the MoO 3 layer through sputtering and thermal evaporation, respectively. The SiO 2 layer acted as a diffusion membrane to control the amount of MoO 3 vapor that broke the SiO 2 layer (Fig. 1b and Supplementary Fig. 2 ), diffused upward and reacted with the NaF layer at a temperature higher than 500 °C to form liquid-phase Na 2 Mo 2 O 7 and gas-phase MoO 2 F 2 (Fig. 1b and Supplementary Fig. 3 ). Simultaneously, the consumption of NaF generated holes and pathways in the NaF layer, which allowed Na 2 Mo 2 O 7 and MoO 2 F 2 to gradually rise to the top surface of the NaF through the pressure gradient and capillary phenomenon (Fig. 1c ). Meanwhile, sulfur vapor was introduced into the system and rapidly dissolved in the eutectic liquid (Na 2 Mo 2 O 7 ) that rose to the surface. As discussed in the first VLS paper, the products of this VLS reaction were MoS 2(s) and sulfur oxides (SO 2(g) and SO 3(g) ) [30] . Moreover, the molten liquid surface provided a temporarily atomic-flat and defection-free surface with a low nucleation density [23] , [32] . The oversaturated MoS 2 precipitated as seed layers on the liquid surface (Fig. 1e ). The as-formed MoS 2 seed layers blocked the route for sulfur to dissolve into the liquid and redirected the underlying liquid to move horizontally. The unsaturated liquid then emerged to the surface at the MoS 2 edge, and this was where the SCVLS reaction primarily occurred. Therefore, MoS 2 laterally grew into large crystals (Fig. 1f , g ). Millimeter-sized MoS 2 single crystals were obtained using this SCVLS method. The large triangular MoS 2 flakes are single crystals in nature, as validated by diffraction analysis at multiple spots in a large flake (Supplementary Fig. 4 ). The zoom-in image of a MoS 2 edge exhibits many bilayer fringes (Fig. 1h ), which were a result of the precipitation of the residual liquid at the edges of the MoS 2 flakes during the rapid cooling process. These fringes validate the existence of the liquid phase during growth and the aforementioned mechanism. In contrast to the conventional CVD method, wherein the nonuniform gas flow in the furnace often gives resultant film of poorer uniformity [33] , extending the SCVLS method to a wafer scale is facile because the precursor rises uniformly from the bottom surface of the growth substrate. Supplementary Fig. 5 shows a full-coverage MoS 2 film grown on a sapphire of 3 × 3 cm 2 (size was only limited by the CVD tube size). This process can also be extended to grow MoSe 2 by replacing sulfur with selenium, result of which is shown in Supplementary Fig. 6 . Fig. 1: Schematics of SCVLS growth mechanism and the grown MoS 2 . a Structure of the solid precursor used for the SCVLS method. b At growth temperature, MoO 3 vaporized and penetrated through the SiO 2 diffusion membrane. MoO 3 and NaF reacted to form liquid-phase Na 2 Mo 2 O 7 (colored in red) at the growth temperature. c Through reactive digging and the capillary effect, the liquid precursor gradually rose to the NaF matrix surface. d Sulfur vapor was introduced into the system and started to dissolve into the Na 2 Mo 2 O 7 liquid. e Liquid precursor sulfurized into the MoS 2 seed layer. f Capped by the MoS 2 , the emerging liquid was redirected horizontally and converted into MoS 2 when it contacted and dissolved sulfur vapor at the edge of the MoS 2 flakes. g A 1-mm MoS 2 flake grown through the SCVLS method. Scale bar is 200 µm. h Magnified image of the MoS 2 grain edge. The fringes at the edge indicate the presence of the liquid precursor during the growth process. Scale bar is 20 µm. Full size image Characterization of as-grown material Compared with the conventional CVD technique, the final products of this SCVLS method were more complex (Fig. 2a ), which comprised two parts: the top MoS 2 layer and the complex solid products generated by the quenched liquid within the NaF matrix. During the sulfurization process, sulfur vapor was primarily dissolved into the liquid through the exposed liquid–gas interface, and thus, the oversaturated liquid could continuously precipitate MoS 2 at the edge of the MoS 2 seeds. However, the reactions were not limited to the top surface. With a lower sulfur concentration, some incomplete sulfurization reactions and precipitations were observed within the NaF matrix (Supplementary Fig. 7 ). Upon cooling, the unsaturated liquid solidified and resided below the MoS 2 flakes or was buried in the NaF matrix (Fig. 2a ). X-ray photoelectron spectroscopy (XPS) was used to analyze the final products. Figure 2b, c shows Mo-3 d and S-2 p spectra obtained from regions covered by large MoS 2 flakes and regions with the exposed NaF matrix, respectively. 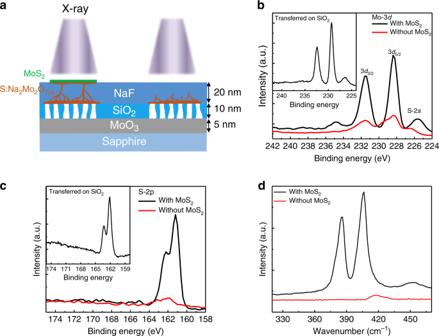Fig. 2: Characterization of the MoS2monolayer and remaining solid precursors. aSchematic of the sampling areas of XPS. XPS data ofbMo-3dandcS-2pon sites that were covered (black) and not covered (red) with MoS2. The broad peak of Mo-3dat sites that were not covered with MoS2indicates the complex chemical environment of Mo below the surface. Insets inbandcare the Mo-3dand S-2pof the MoS2film transferred onto a SiO2substrate.dRaman spectra taken form positions with (black) and without (red) MoS2coverage. For a region covered with MoS 2 , the Mo-3 d peak of ~230–228 eV could be deconvoluted into sharp Mo 4+ and broad Mo x + . The Mo 4+ signal was obtained from the top MoS 2 , and the Mo x + signal was obtained from the precipitates and solidified liquid phase in the NaF matrix, as shown using an XPS depth profile (Supplementary Fig. 7 ). With a lower sulfur concentration in the matrix, the possible products for the precipitate and quenched liquid were amorphous MoS 2 , MoO 2 , and MoS x O y , comprising the Mo x + signal. In addition, a small peak at ~235 eV indicates Mo 6+ , which is the peak from Na 2 Mo 2 O 7 , indicating the presence of residual unreacted precursor below MoS 2 ; this supports the as-proposed horizontal transport of the liquid. For a region without MoS 2 , only a small amount of sulfur diffused into the NaF matrix and reacted with the liquid below the surface. Figure 2b, c shows a considerably weaker Mo x + and sulfur signal, which indicates that no liquid rose to the top surface. The resultant products were further characterized using Raman spectroscopy (Fig. 2d ). The region covered with MoS 2 exhibited sharp E 2g and A 1g peaks with a spacing of 19.5 cm −1 , thus validating the high quality and monolayer characteristics for the as-grown MoS 2 . The region that was not covered by MoS 2 exhibited no significant Raman signal, which validated the absence of any crystalline product in the NaF matrix. The as-grown monolayer MoS 2 could be readily transferred to various substrates using the conventional polymethyl-methacrylate (PMMA) method. Atomic force microscopy images and photoluminescence spectrum in Supplementary Fig. 8 and 9 also confirm the monolayer property. The insets of Fig. 2b, c show the XPS results of the as-transferred MoS 2 on silica. Compared with the as-grown sample, the transferred MoS 2 exhibited sharp and clean Mo 4+ signals at 229.3 and 232.4 eV. The Mo–S ratio, which was calculated by integrating the area of the Mo and S signals, was 1:2, as expected for high-quality MoS 2 . Fig. 2: Characterization of the MoS 2 monolayer and remaining solid precursors. a Schematic of the sampling areas of XPS. XPS data of b Mo-3 d and c S-2 p on sites that were covered (black) and not covered (red) with MoS 2 . The broad peak of Mo-3 d at sites that were not covered with MoS 2 indicates the complex chemical environment of Mo below the surface. Insets in b and c are the Mo-3 d and S-2 p of the MoS 2 film transferred onto a SiO 2 substrate. d Raman spectra taken form positions with (black) and without (red) MoS 2 coverage. Full size image Controlling the coverage and thickness of MoS 2 With a suitable sulfur source, the growth rate of SCVLS process was controlled by horizontal transport rate of the liquid. Rapid horizontal mass transport of the liquid was crucial for growing large monolayer MoS 2 . The driving force stemmed from the diffusion and capillary phenomena of the high-pressure liquid and gas produced by the eutectic reaction (Fig. 3a ). Because MoS 2 layers covered the top surface and confined the liquid flow, the vertical driving force was redirected horizontally, and both vertical and horizontal liquid transport was promoted with increasing amount of liquid source. The rapid SCVLS reaction could thus be performed under this condition, and the rapid growth rate abruptly increased the grain size of MoS 2 . However, when the driving force was weak, the low growth rate would result in more nucleation seeds on NaF, thus reducing the average size of the MoS 2 crystals. In some regions, the weak driving force was not sufficient to push the liquid to the surface. The sulfur vapor would slowly diffuse into the NaF matrix, react with the liquid, and eventually solidify. Therefore, no MoS 2 was grown on the surface under this condition, and this phenomenon reduced the coverage of MoS 2 . Here, the vertical driving force was controlled using different amounts of MoO 3 sources. Figure 3b–d shows the optical images of the as-grown MoS 2 with different thicknesses of MoO 3 precursor layers. 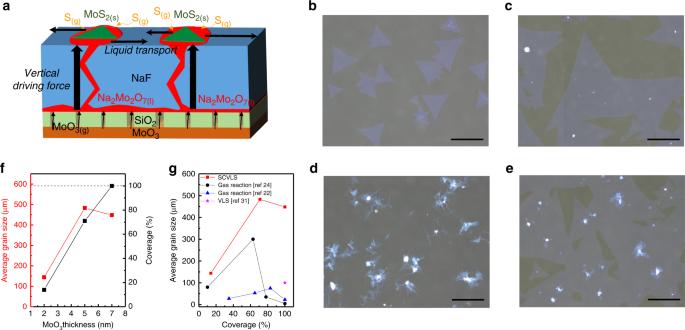Fig. 3: Driving forces of SCVLS reaction. aSchematic of the vertical driving force and horizontal liquid transport. Optical microscopy images of MoS2grown usingb2-nmc5-nm, andd7-nm MoO3as a solid precursor. The growth time was 10 min.e1-min growth using the same precursor sample as ind. The scale bars inb,d, andeare 200 µm and the one incis 300 µm.fAverage grain size and coverage of the MoS2flakes as a function of MoO3precursor thickness.gComparison of SCVLS, VLS, and gas-phase CVD. SCVLS reaction enables a relatively large-grain size when a full-coverage film was achieved. The grain size and coverage of MoS 2 abruptly increased with the increasing thickness of MoO 3 precursor (Fig. 3f ). In order to estimate the grain size of the full-coverage film (Fig. 3d ), the growth time was reduced from 10 (Fig. 3d ) to 1 min (Fig. 3e ), to monitor the grain size before grains merged into continuous film. The average grain size of the full-coverage film was ~450 µm, which is the largest recorded average grain size for completely covered MoS 2 film. Although there are some thick islands on the film (Fig. 3d and Supplementary Fig. 10 ), this large-grain continuous film can still demonstrate outstanding electrical performance shown in the later section. The trend of the coverage and average grain size versus the precursor thickness in SCVLS (Fig. 3f ) is very different from that for the common gas-phase reaction CVD. For gas-phase CVD, the average grain size of the continuous film is reduced by a factor of 10–100 compared with the largest isolated crystals because the larger amount of the precursor for growing continuous film abruptly led to the increased nucleation density and thus reduced grain size (Fig. 3g ) [25] , [34] . However, for SCVLS method, the average grain sizes of the continuous film (450 µm) and largest isolated crystals (500 µm) are similar because of the self-capping effect and the fast transport of liquid. Furthermore, coverage of ~82% was reached within 1 min of fabrication (Fig. 3e ), which demonstrates the rapid growth rate (370 µm/min, see Supplementary Fig. 11 ). This may be a result from the fast transport of liquid assisted by the fluoride surface, which has been shown to enhance growth rate of 2D materials [35] . The driving force and nucleation density could be further controlled by tuning the thickness of SiO 2 membranes, growth temperature, and the thickness of NaF (Supplementary Figs. 12 – 14 ). Fig. 3: Driving forces of SCVLS reaction. a Schematic of the vertical driving force and horizontal liquid transport. Optical microscopy images of MoS 2 grown using b 2-nm c 5-nm, and d 7-nm MoO 3 as a solid precursor. The growth time was 10 min. e 1-min growth using the same precursor sample as in d . The scale bars in b , d , and e are 200 µm and the one in c is 300 µm. f Average grain size and coverage of the MoS 2 flakes as a function of MoO 3 precursor thickness. g Comparison of SCVLS, VLS, and gas-phase CVD. SCVLS reaction enables a relatively large-grain size when a full-coverage film was achieved. Full size image In addition to large-grain continuous film, layer-controlled growth of bilayer and multilayer are also attractive because of the better electrical performance of few-layer MoS 2 [36] , [37] , [38] , [39] . SCVLS can also control the layer number of MoS 2 with its special growth mechanism we proposed. In the growth condition of previous paragraphs, sulfur vapor was introduced before or during the liquid’s rise to the surface. The small liquid droplets rapidly dissolved sulfur and formed monolayer MoS 2 capping seeds, which promoted the horizontal mass transport and formed large monolayer MoS 2 grains. It is noteworthy to mention that the SCVLS reaction can be dynamically controlled by changing the timing of sulfurization (Fig. 4a ). When sulfur vapor was introduced later, the emerged liquid would form into a large droplet (Supplementary Fig. 15 ). During sulfurization, the as-formed small MoS 2 seeds were buried in the oversaturated liquid. Under this condition, fresh MoS 2 could be formed at the edge of the original seeds, and a second layer could be grown on the MoS 2 seeds (Fig. 4b ). Large bilayer MoS 2 crystals could be fabricated by delaying the sulfurization timing for 2 min. Trilayer MoS 2 was occasionally observed when sulfurization is delayed. Figure 4c–e are the optical images of the transferred mono-, bi-, and trilayer MoS 2 on SiO 2 /Si substrates, respectively. 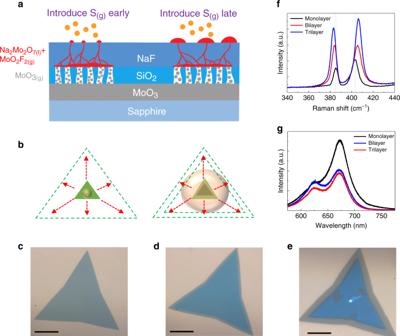Fig. 4: Dynamic effect on SCVLS method. aSchematic of the timing of introducing sulfur vapor affecting the final growth product.bWhen sulfur vapor was introduced early, the Na2Mo2O7precursor rapidly formed the MoS2seed layer when exposed on the surface (left). When sulfur vapor was introduced later, the MoS2seed layer was formed at the solid–liquid interface, thus leaving a droplet of the liquid precursor on top of the interface. This droplet was later sulfurized into the second layer of MoS2(right). Optical images of the transferredcmonolayer,dbilayer, andetrilayer MoS2. Scale bars are 50 µm.fRaman andgphotoluminescence spectra of the monolayer, bilayer, and trilayer MoS2. The clear optical contrast shows the characteristics of the mono-, bi-, and trilayers of each MoS 2 . AFM images in Supplementary Fig. 16 also confirm the thickness of these samples. Figure 4d, e shows that the second and third layers are well-aligned with the bottom MoS 2 layer, thus indicating the epitaxial growth of an excess MoS 2 layer. The diffraction patterns manifest a 2H-type stacking order of the SCVLS reaction (Supplementary Fig. 17 ) [30] . Raman spectra in Fig. 4f further validate the layer number and strong interaction between the mono-, bi-, and trilayer MoS 2 grown using the SCVLS method. The peak separations of E 2g and A 1g are 18.0, 21.5, and 23.2 cm −1 , which are similar to the values previously reported for exfoliated MoS 2 [40] . The strong interaction between each layer changes the dielectric environment, thus softening the in-plane E 2g mode (red-shift). Moreover, the strong interaction between interlayer S increases the restoring force, thus stiffening the out-of-plane A 1g mode (blue shift) [40] . The photoluminescence spectra in Fig. 4g exhibit clear quenched signals for bilayer and trilayer MoS 2 because of the direct–indirect band gap transition for monolayer and bilayer MoS 2 [4] , [6] . By employing dynamic control of sulfurization, a large bilayer single crystal (200 µm) is successfully synthesized, the grain size of which is comparable to the large bilayer crystals in the previous studies [37] , [38] . Moreover, the ability to change the layer number of MoS 2 by controlling the size of the droplet validated the SCVLS mechanism proposed in Fig. 1 . Fig. 4: Dynamic effect on SCVLS method. a Schematic of the timing of introducing sulfur vapor affecting the final growth product. b When sulfur vapor was introduced early, the Na 2 Mo 2 O 7 precursor rapidly formed the MoS 2 seed layer when exposed on the surface (left). When sulfur vapor was introduced later, the MoS 2 seed layer was formed at the solid–liquid interface, thus leaving a droplet of the liquid precursor on top of the interface. This droplet was later sulfurized into the second layer of MoS 2 (right). Optical images of the transferred c monolayer, d bilayer, and e trilayer MoS 2 . Scale bars are 50 µm. f Raman and g photoluminescence spectra of the monolayer, bilayer, and trilayer MoS 2 . Full size image High-performance FET device The electrical properties of the large monolayer MoS 2 crystal grown by the SCVLS method was examined by measuring the transport properties of MoS 2 FETs. Figure 5a shows an FET with a back-gate structure and 90-nm-thick SiO 2 . 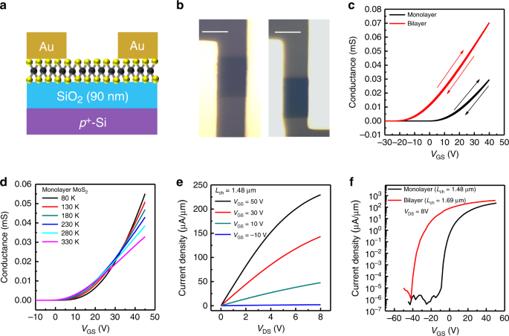Fig. 5: Transport properties of the MoS2grown through the SCVLS method. aSchematic image of a back-gate monolayer MoS2transistor.bOptical image of a monolayer and bilayer FETs. Both scale bars are 5 µm.cGate-dependent conductance of devices shown inb.dTemperature-dependent transport property of the monolayer MoS2FET shown inb. A clear MIT is observed atVGSof 30 V.eVDS-dependent source-drain current density of the monolayer device at different gate voltages. The channel length is 1.48 μm.fLog plot of the gate-dependent current density of the short channel mono- and bilayer devices under an 8-V source-drain bias. The on/off ratio is 5 × 108. Both mono- and bilayer MoS 2 FETs were fabricated as shown in Fig. 5b and Supplementary Fig. 18 . Figure 5c displays the gate-dependent conductance of the MoS 2 FETs. Both devices have a very small hysteresis, indicating low defect and impurity induced trap density in the SCVLS growth and the device fabrication processes. The field-effect mobility was calculated using \(\mu _{FE} = \frac{{L_{CH}}}{W}\frac{1}{{C_G}}\frac{{dG}}{{dV_{GS}}}\) , where C G , L CH , W , V GS , and G stand for the back-gate capacitance, channel length, channel width, back-gate voltage, and sheet conductance of the channel, respectively. Because of its higher carrier density and stronger charge screening effect, bilayer MoS 2 has a smaller threshold voltage ( V th ) and higher mobility. The mobilities of the mono- and bilayer MoS 2 FETs are 33 and 49 cm 2 V −1 S −1 , respectively. These values are comparable to the exfoliated MoS 2 [41] and the best reported values of CVD MoS 2 on SiO 2 [38] , [42] , [43] , showing the high quality of MoS 2 grown through the SCVLS method. The temperature-dependent transport also confirms the quality of SCVLS MoS 2 as shown in Fig. 5d . For the monolayer device, a clear metal–insulator transition (MIT) was observed, which is generally detected when using a high- k dielectric layer to reduce Columbic scattering in the MoS 2 channel [2] . For back-gate devices without a high- k dielectric layer, a clear MIT occurs only when using high-quality MoS 2 with a low concentration of sulfur vacancies. In general, according to the Ioffe-Regel criterion [44] , MIT occurs when the critical channel conductance is approximately one quantum conductivity ( e 2 / h ) [2] , [44] . If the crossover point is in a lower carrier concentration region, this directly reflects the high-mobility property of MoS 2 [45] , [46] . The carrier concentration of the transition point is calculated using 
    n_MIT = C_G/e( V_T - V_MIT),
 (1) where V T and V MIT are the threshold voltage and voltage at which the MIT occurs, respectively [47] , [48] . The n MIT of the SCVLS MoS 2 in this study is 4.3 × 10 12 cm −2 , which is even lower than the previously reported intrinsic exfoliated MoS 2 with low S-vacancy concentration [47] . This indicated the high quality and low sulfur vacancy concentration of the MoS 2 fabricated using the SCVLS method. Figure 5e is the output characteristics of a short channel (1.48 μm, see Supplementary Fig. 19 ) monolayer FET at various back-gate voltages. 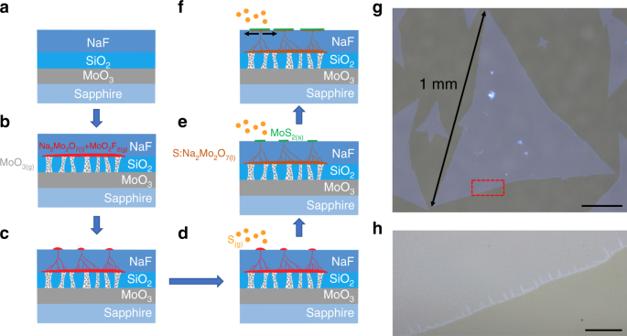The linear behavior in the low source-drain voltage ( V DS ) region shows a good Ohmic property of contacts. Figure 5f presents the semi-logarithmic of the gate-controlled current density. The device on/off ratio can reach 5 × 10 8 , with a subthreshold swing of 980 mV dec −1 . The maximum current density in the monolayer MoS 2 is 230 µA µm −1 (390 μA μm −1 for bilayer), potentially comparable to the optimal reported in consideration of the difference in contact geometry [38] , [42] . Fig. 1: Schematics of SCVLS growth mechanism and the grown MoS2. aStructure of the solid precursor used for the SCVLS method.bAt growth temperature, MoO3vaporized and penetrated through the SiO2diffusion membrane. MoO3and NaF reacted to form liquid-phase Na2Mo2O7(colored in red) at the growth temperature.cThrough reactive digging and the capillary effect, the liquid precursor gradually rose to the NaF matrix surface.dSulfur vapor was introduced into the system and started to dissolve into the Na2Mo2O7liquid.eLiquid precursor sulfurized into the MoS2seed layer.fCapped by the MoS2, the emerging liquid was redirected horizontally and converted into MoS2when it contacted and dissolved sulfur vapor at the edge of the MoS2flakes.gA 1-mm MoS2flake grown through the SCVLS method. Scale bar is 200 µm.hMagnified image of the MoS2grain edge. The fringes at the edge indicate the presence of the liquid precursor during the growth process. Scale bar is 20 µm. Table 1 lists the recently reported monolayer MoS 2 back-gate FETs. MoS 2 grown by the SCVLS method exhibits the largest grain size and remarkable electrical performance compared with other CVD techniques. The good uniformity of the large monolayer crystal is confirmed by measuring 18 FETs in a 1-mm crystal (Supplementary Fig. 20 ). In addition, with the capability of growing large-grain and continuous film, we fabricated hundreds of devices across a 1.5 × 1.5-cm area, as shown in Fig. 6a, b . 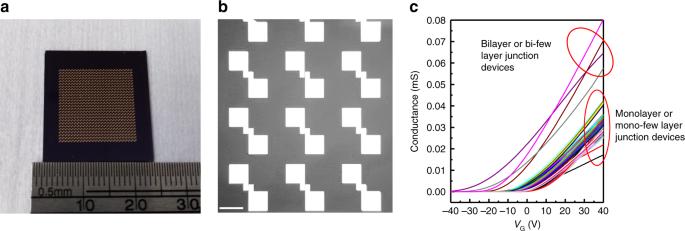Fig. 6: Transport properties of the large-grain, continuous film. aPhoto-image of the as-fabricated FETs across a 1.5 × 1.5-cm region.bOptical image of FET devices. The scale bar is 150 μm. The fine feature is shown in Supplementary Fig.18.cGate-dependent conductance of the devices across the large area. Figure 6c is the gate-dependent conductance of a hundred devices in the whole area. Ninety percent of devices have pure monolayer channel and show high mobilities (34 ± 7 cm 2 V −1 s −1 ) with small variation of V th (4.9 ± 2.3 V). Devices have larger variation in mobility and V th if their channels are bilayer, few-layer, mono-few-layer junction, or monolayer with a small few-layer flake on top. However, the mobilities are still high for all of the devices because of the large-grain monolayer underneath (Supplementary Fig. 21 ). This demonstrates the advantage of using the SCVLS method for practical applications. Fig. 5: Transport properties of the MoS 2 grown through the SCVLS method. a Schematic image of a back-gate monolayer MoS 2 transistor. b Optical image of a monolayer and bilayer FETs. Both scale bars are 5 µm. c Gate-dependent conductance of devices shown in b . d Temperature-dependent transport property of the monolayer MoS 2 FET shown in b . A clear MIT is observed at V GS of 30 V. e V DS -dependent source-drain current density of the monolayer device at different gate voltages. The channel length is 1.48 μm. f Log plot of the gate-dependent current density of the short channel mono- and bilayer devices under an 8-V source-drain bias. The on/off ratio is 5 × 10 8 . Full size image Table 1 Comparison of the different CVD methods. Full size table Fig. 6: Transport properties of the large-grain, continuous film. a Photo-image of the as-fabricated FETs across a 1.5 × 1.5-cm region. b Optical image of FET devices. The scale bar is 150 μm. The fine feature is shown in Supplementary Fig. 18 . c Gate-dependent conductance of the devices across the large area. Full size image In summary, a new concept of growing high-quality single-crystal 2D materials from the liquid precursor was proposed using the SCVLS method. The rapid horizontal mass transport promotes the lateral growth of 2D materials and allows the growth of MoS 2 flakes as large as 1.1 mm. The self-capping effect drastically reduces the nucleation density even under large amount of precursor and results in a wafer scale, 100% coverage MoS 2 films with an average grain size of up to 450 µm. It overcomes the bottleneck of the conventional gas-phase CVD reaction, which is the trade-off between coverage and grain size. The quality and uniformity of the as-grown MoS 2 were carefully evaluated through the electrical properties of MoS 2 FETs across a large area. High-mobility MoS 2 devices are demonstrated across a 1.5 × 1.5-cm area. Moreover, this method is capable of fabricating large bilayer MoS 2 crystals by controlling the timing of sulfurization. More sophisticated sulfurization precursor such as H 2 S is expected to improve the layer number control or the uniformity of continuous films. Fabricating crystals by using the liquid–solid reaction, such as in doping and alloying, is one expected niche of this SCVLS method, which provides a new approach for synthesizing industrial-grade 2D materials for practical applications in 2D electronics. Preparation of solid precursor 3 × 3-cm c-plane (0001) sapphire substrate was cleaned first by deionized water then sonicated in acetone and isopropyl alcohol for 20 and 5 min, respectively. MoO 3 film with well-controlled thickness was grown on top of sapphire substrates with a homemade PEALD system using Mo(CO) 6 as precursor and oxygen plasma as the oxidation reactant. For each deposition cycle, a Mo(CO) 6 precursor pulse is provided into the chamber, then the excess precursor is purged away by argon, and finally oxygen plasma (up to 200 W) is used to oxidize the precursor and form uniform MoO 3 film. Thermal evaporation can be used to replace the PEALD process for depositing MoO 3 but will result in worse MoS 2 morphology (Supplementary Fig. 22 ). SiO 2 film was deposited on top of MoO 3 layer by sputtering a 3-inch SiO 2 target with Ar plasma at a power density of 0.6 W/cm 2 in a radio-frequency magnetron sputtering system. NaF thin film was deposited onto the sample by heating NaF powder (Acros, 97%) loaded in a Mo boat in a high vacuum evaporator chamber (<5 × 10 −5 torr). For sputtering and thermal evaporation film, film thickness was monitored by a quartz crystal microbalance and the deposition rate was maintained at 0.1 Ås −1 . Samples were attached to a spinning sample holder to obtain high uniformity. Growth of MoS 2 High temperature growth was carried out in a 2-inch quartz tube and the temperature profile of the growth was controlled by a three-zone furnace. Sulfur powder (Aldrich, 99.98%), which was placed in an alumina crucible, and precursor sample held by a 3 × 3-cm 2 quartz plate were placed at the center of first and third hearing zone, respectively, as depicted in Supplementary Fig. 1 c. A 5 sccm H 2 and 50 sccm Ar mixed gas flow was used as carrier gas and the pressure within the quartz tube was controlled to be 30 torr. The temperature at the sample ramped up at a rate of 40 °C min −1 to 800 °C and was held for 10 min. Sulfur vapor was introduced by ramping up the temperature at the first zone at a rate of 15 °C min −1 and was held at the desired temperature during growth. After growth, the furnace was turned off and was fast-cooled using an industrial fan. The temperature ramping profile is shown in Supplementary Fig. 1d . For monolayer MoS 2 growth, A and B setpoints are reached at the same time. For bilayer MoS 2 growth, the B setpoint is reached 2 min later than the A setpoint. Device fabrication and characterization p -type heavily doped silicon wafers with 90-nm thermal oxide layers were used for back-gate FET devices. MoS 2 films/isolated crystals were transferred to wafers through a conventional PMMA method. Optical lithography and oxygen plasma were used to define the MoS 2 strips. Then, the second lithography process defined the source-drain patterns. A 50-nm gold layer was thermally evaporated under high vacuum as the source-drain and back-gate electrodes. Before measuring electrical properties, FETs were annealed at 120 °C under a 10 −3 torr vacuum for 10 h in a probe station (Lakeshore). Gate and source-drain voltage were applied by Kethley 6487 picometers. Raman and photoluminescence spectra were measured by a confocal system equipped with a 476-nm laser. XPS spectra were obtained using PHI VersaProbe system. Transmission electron analysis (Supplementary Figs. 4 , 17 , and 23 ) was performed in JEOL AEM 2010F and JEOL AEM 2100F, which was equipped with a probe-type corrector for the spherical aberration of the objective lens. Both systems were operated at 200 kV for the analysis.